Spherical trihedral metallo-borospherenes The discovery of borospherenes unveiled the capacity of boron to form fullerene-like cage structures. While fullerenes are known to entrap metal atoms to form endohedral metallofullerenes, few metal atoms have been observed to be part of the fullerene cages. Here we report the observation of a class of remarkable metallo-borospherenes, where metal atoms are integral parts of the cage surface. We have produced La 3 B 18 – and Tb 3 B 18 – and probed their structures and bonding using photoelectron spectroscopy and theoretical calculations. Global minimum searches revealed that the most stable structures of Ln 3 B 18 – are hollow cages with D 3 h symmetry. The B 18 -framework in the Ln 3 B 18 – cages can be viewed as consisting of two triangular B 6 motifs connected by three B 2 units, forming three shared B 10 rings which are coordinated to the three Ln atoms on the cage surface. These metallo-borospherenes represent a new class of unusual geometry that has not been observed in chemistry heretofore. The electron deficiency of boron often leads to electron delocalization and the violation of the octet rule in boron compounds and three-dimensional (3D) cage units in different bulk boron allotropes [1] , [2] , [3] . Because of the strong boron–boron bonding, there were speculations about the formation of boron nanotubes composed of a triangular boron lattice [4] , [5] , after the discovery of carbon nanotubes. The triangular boron lattice can be viewed as a graphene-like sheet with the filling of a boron atom in each B 6 hexagon. Further theoretical calculations revealed, however, that triangular lattices with hexagonal vacancies were more stable and more suitable to construct boron nanotubes [6] , [7] . In the meantime, combined spectroscopic and theoretical studies have shown that size-selected boron clusters all have 2D structures with delocalized multi-center bonding within the cluster plane [8] , [9] , [10] , [11] . The discovery of the hexagonal 2D B 36 clusters provided the first experimental evidence of the viability of atom-thin boron nanostructures with hexagonal vacancies, named as borophene akin to graphene [12] . Borophenes have been recently synthesized using atomic vapor deposition on Ag(111) substrates [13] , [14] , forming a new class of synthetic 2D nanomaterials [15] . The analogy between nanostructures made of boron and carbon has been further extended when the B 40 and B 39 – clusters were found to have global minimum cage structures [16] , [17] , i.e. borospherenes analogous to the fullerenes. Fullerenes are known to form endohedral metallofullerenes for alkali, alkali earth, lanthanide, and actinide elements [18] , [19] , albeit not for transitions metals. Heterofullerenes in which one carbon atom is substituted by a transition metal atom have been observed in the gas phase, but the metal substitution induces large local structural distortions and such heterofullerenes have not been synthesized in the bulk [20] , [21] , [22] . The first cage cluster made of multiple metal atoms and carbons was proposed to be Ti 8 C 12 + (metallocarbohedrene) [23] . However, subsequent theoretical calculations showed that the metallocarbohedrene is not stable and the global minimum of Ti 8 C 12 + consisted of a tetrahedral, close-packed Ti 8 clusters coordinated by six C 2 units on the cluster surface [24] . In the present article, we report the first observation of a class of metallo-borospherenes, hollow cage clusters consisting of three lanthanide (Ln) atoms and 18 boron atoms (Ln 3 B 18 – ). Transition-metal-doped boron clusters were first found to form aromatic borometallic molecular wheels, M©B n − ( n = 8–10) [25] , [26] , as well as metal-centered nanotubular structures [27] . More interestingly, it has been shown that transition metals can be an integral part of larger 2D boron clusters [28] , leading to the possibility of metallo-borophenes [29] . Lanthanide-doped boron clusters, however, have been found recently to form very different structures, due to both charge transfer interactions and strong ( d–p ) π bonding [30] . For example, lanthanide-doped boron clusters do not form similar borometallic molecular wheels as the transition metals. Instead, they form inverse-sandwich-type structures for Ln 2 B n – clusters ( n = 7–9) [31] , [32] . The most recent study indicates that the inverse-sandwich structure may extend to form lanthanide-boron nanowires [33] . Here we report a joint photoelectron spectroscopy (PES) and quantum chemistry study of two tri-lanthanide-doped B 18 clusters (La 3 B 18 – and Tb 3 B 18 – ), which are found to possess unprecedented D 3 h cage structures with the Ln atoms being integral parts of the cage surface. These D 3 h metallo-borospherenes belong to an unusual class of geometry known as spherical trihedron. The B 18 framework consists of two B 6 triangles connected by three B 2 units, forming three shared B 10 rings. The high stability of the spherical trihedral structures is derived from the strong interactions between the Ln atoms and the B 10 rings via charge transfer interactions and d – p covalent bonding. Theoretical calculations show that the entire series of lanthanide elements (Ln = La–Lu) can form spherical trihedral Ln 3 B 18 – metallo-borospherenes with tunable magnetic properties, making them a fascinating series of building blocks for new types of magnetic materials. Photoelectron spectroscopy The PE spectrum at 193 nm was first measured for the La 3 B 18 – cluster (Fig. 1a ), which was found to exhibit a relatively simple pattern compared with that of the recently reported La 3 B 14 – cluster [33] . This observation suggested that La 3 B 18 – should possess a highly symmetric structure. Subsequently, we also obtained the spectrum of a late-Ln cluster Tb 3 B 18 – (Fig. 2a ) and observed a spectral pattern, exhibiting some similarities to that of La 3 B 18 – and suggesting that these two Ln-doped boron clusters should have similar structures and chemical bonding. The well-resolved PES features of the Ln 3 B 18 – clusters serve as electronic fingerprints to allow analyses of their structures and chemical bonding by comparing with theoretical calculations, as shown in Figs. 1 b, 2b , and Supplementary Tables S1 and S2 for Ln = La and Tb, respectively. Fig. 1: Photoelectron spectrum of La 3 B 18 – . a At 193 nm. b The simulated spectrum. Full size image Fig. 2: Photoelectron spectrum of Tb 3 B 18 – . a At 193 nm. b The simulated spectrum. Full size image The spectrum of La 3 B 18 – displayed five well-resolved bands labeled as X, A, B, C, and D (Fig. 1a ). The X band yielded the first vertical detachment energy (VDE) of 2.97 eV for La 3 B 18 – . The adiabatic detachment energy (ADE) for band X was evaluated from its onset to be 2.80 eV, which also represents the electron affinity (EA) of neutral La 3 B 18 . The higher binding energy bands (A, B, C, and D) correspond to detachment transitions to the excited states of neutral La 3 B 18 . The A band at 3.64 eV was broad and not well resolved at 193 nm, but it was slightly better resolved in the 266 nm spectrum (Supplementary Fig. 1 ). This broad spectral feature could be due to geometry changes upon electron detachment or overlapping detachment transitions. Band B at 4.01 eV is sharper compared with band A (Fig. 1a ). An intense and sharp band C at 4.43 eV was clearly resolved in the 193 nm spectrum. Following a large energy gap, a broad band (D) was observed above ~5.5 eV. Due to the poor signal-to-noise ratio, band D was tentatively assigned for the sake of discussion. The PE spectrum of Tb 3 B 18 – showed five well-resolved peaks assigned as X, A, B, C, D (Fig. 2a ). The X band gave rise to a VDE of 3.26 eV for Tb 3 B 18 – and an ADE of 3.13 eV, which is also the EA of neutral Tb 3 B 18 . Band A was observed at a VDE of 3.84 eV, followed by three closely-lying bands (B, C, D). Band B at 4.28 eV and band C at 4.52 eV were relatively weak and closely spaced, whereas band D at 4.77 eV was much more intense. Beyond ~5 eV, the signal-to-noise ratio was poor and no obvious spectral bands were observed. Band E close to the threshold at a VDE of ~6.2 eV was tentatively labeled. The overall spectral pattern for Tb 3 B 18 – exhibits some similarity to that of La 3 B 18 – . In particular, the strong X and D bands in Tb 3 B 18 – are similar to the strong X and C bands in La 3 B 18 – . There is a large energy gap on the high binding energy side in both spectra. Similar spectral patterns could be an indication of similar structures, as have been observed for a series of dilanthanide clusters (Ln 2 B 8 – ) [31] . Global minimum structural searches The low-lying isomers within 55 kcal mol −1 of the global minimum at the levels of PBE/TZP and PBE0/TZP are presented in Supplementary Fig. 2 . The global minimum of La 3 B 18 – is a hollow cage with a closed-shell ground state ( 1 A 1 ) and D 3 h symmetry. This is a hetero-metallo-borospherene, in which the three La atoms are integral parts of the cage surface, as shown in Fig. 3 . All the other low-lying isomers are low-symmetry 3D structures, many of which are distorted cages. The highly symmetric global minimum D 3 h metallo-borospherene exhibits overwhelming stability relative to the other low-lying isomers: it is more stable than the nearest isomer with C s symmetry by ~19 kcal mol −1 at the PBE/TZP and PBE0/TZP levels of theory. The B 18 framework in the La 3 B 18 – cage can be viewed as consisting of two B 6 triangles linked together at their three corners by three B 2 units, creating three shared B 10 rings along the C 3 axis. The three La atoms are coordinated by the three B 10 rings, giving rise to the closed cage structure. The La 3 B 18 – metallo-borospherene has an oblate shape with a diameter of 4.62 Å along the C 3 axis (between the two B 6 triangles) and 5.09 Å encompassed by the three equatorial La atoms. The relevant bond lengths of the La 3 B 18 – metallo-borospherene are shown in Supplementary Fig. 3a . Fig. 3: The global minimum structure of La 3 B 18 – ( D 3 h , 1 A 1 ) at the PBE0/TZP level. a The C 3 axis is along the page vertically. b The C 3 axis is perpendicular to the page. Full size image The hollow cage structure of La 3 B 18 – was totally unexpected and the geometry is highly unusual. To further examine its stability and robustness, we performed ab initio molecular dynamics (AIMD) simulations at different temperatures, 300, 500, 700, and 1000 K (see Supplementary Fig. 4 ). We found that even at 1000 K the La 3 B 18 – metallo-borospherene is dynamically stable for the 13 ps duration of the simulations. At 1000 K, the structure displayed a root-mean-square-deviation of 0.199 Å and a maximum bond length deviation of 0.260 Å during the simulations. The similarity in their PE spectra suggested that the global minima of Tb 3 B 18 – and La 3 B 18 – should be similar. Because of the localized and nonbonding nature of the 4 f orbitals in Tb, we optimized the D 3 h structure for Tb 3 B 18 – using the 4 f -in-core pseudopotential [34] . The structural parameters of the Tb 3 B 18 – metallo-borospherene are similar to those for La 3 B 18 – (Supplementary Fig. 3 ), except that the Tb–B and B–B bond lengths are all slightly shorter due to the smaller atomic radius of Tb as a result of the lanthanide contraction. Because of the use of the 4 f -in-core pseudopotential, the spin state of the Tb 3 B 18 – metallo-borospherene was not determined from the geometry optimization. We performed broken symmetry calculations and compared the relative energies between the ferromagnetic and antiferromagnetic couplings of the 4 f electrons, as shown in Supplementary Table 3 for Tb 3 B 18 – , as well as for Pr 3 B 18 – . The relative energies due to the inter-atomic spin couplings of the unpaired 4 f electrons are relatively small, although the high spin ferromagnetic coupling seems to give the lowest energy in both cases. 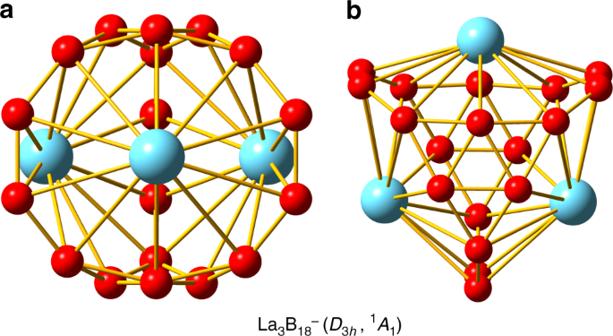Fig. 3: The global minimum structure of La3B18–(D3h,1A1) at the PBE0/TZP level. aTheC3axis is along the page vertically.bTheC3axis is perpendicular to the page. Hence, the spin multiplicity of the Tb 3 B 18 – metallo-borospherene should be 19 (with 18 unpaired 4 f electrons). Comparison between the experimental and theoretical results To validate the D 3 h cage structure for La 3 B 18 – and Tb 3 B 18 – , we calculated their ADEs and VDEs using the ΔSCF–TDDFT formalism. Figures 1 b, 2b present the simulated spectra for the D 3 h global minimum structures, in comparison with the experimental data. The computed ADE/VDE 1 at the CCSD(T) level are 2.828/2.972 eV for La 3 B 18 – (Supplementary Table 4 ), in excellent agreement with the experimental data of 2.80/2.97 eV. As shown in Fig. 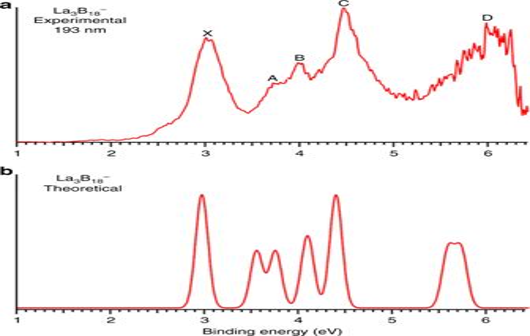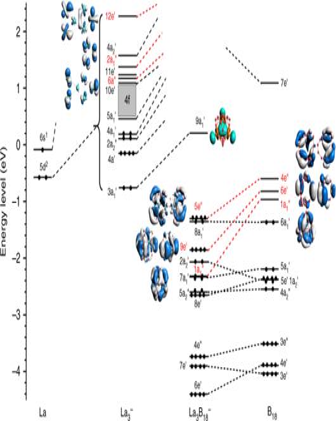Fig. 4: The Kahn–Sham molecular orbital correlation diagram for La3B18–(D3h,1A1). It shows the interactions between the 5dorbitals of the three La atoms and the group orbitals of the B18moiety. 4 , the valence MOs of La 3 B 18 – are mainly of La-B d–p and B sp characters. Fig. 1: Photoelectron spectrum of La3B18–. aAt 193 nm.bThe simulated spectrum. Because La 3 B 18 – has a closed-shell configuration, single-electron removal from each molecular orbital (MO) yields one detachment channel, as shown in Supplementary Table 1 . The computed VDEs for detachment from the 5 e ′′ HOMO (2.972 eV) and 8 a 1 ′ HOMO-1 (2.987 eV) are very close to each other, in excellent agreement with the experimental VDE of the X band (2.97 eV). In fact, each of the observed PES band corresponds to two detachment channels, as given in Supplementary Table 1 , where the electron configurations and final state symmetries are also presented. The simulated spectral patterns and the experimental spectra are in excellent agreement, providing considerable credence for the D 3 h cage global minimum for La 3 B 18 – . We have also simulated the PE spectra for the next nine higher-lying isomers of La 3 B 18 – , as shown in Supplementary Fig. 5 . None of these spectra fits the experimental spectrum, giving additional support for the D 3 h global minimum structure. 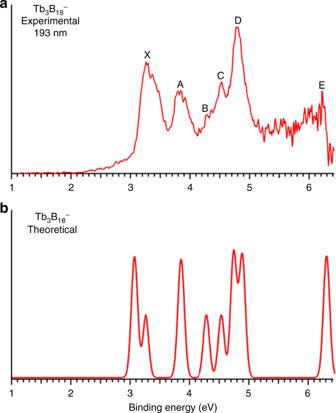The computed ADE/VDE for Tb 3 B 18 – are 2.901/3.017 eV at the CCSD(T) level (Supplementary Table 4 ), slightly underestimated relative to the experimental data of 3.13/3.26 eV probably due to the use of the 4 f -in-core approximation as well as the incomplete account of electron correlations. Nevertheless, the theoretical results by not considering the 4 f electrons and detachment channels are still in very good agreement with the experimental data, as can be seen in Fig. Fig. 2: Photoelectron spectrum of Tb3B18–. aAt 193 nm.bThe simulated spectrum. 2 and Supplementary Table 2 . These results are consistent with our previous observations that the detachment cross sections of the 4 f electrons are much weaker and the PE spectra of Ln–B binary clusters are dominated by the Ln–B d–p and B sp detachment channels [31] , [32] . Fig. 4: The Kahn–Sham molecular orbital correlation diagram for La 3 B 18 – ( D 3 h , 1 A 1 ). It shows the interactions between the 5 d orbitals of the three La atoms and the group orbitals of the B 18 moiety. Full size image Stabilities of the first metallo-borospherenes The observation of the La 3 B 18 – and Tb 3 B 18 – cage clusters, in which the three Ln atoms are integral parts of the cage surface, is unprecedented. The two B 6 triangles in the D 3 h structure are reminiscent of the B 40 borospherene [16] , which consists of eight fused B 6 triangles on a spherical surface. Hence, the Ln 3 B 18 – cage clusters can be viewed as a new class of metallo-borospherenes. Networked metallo-fullerenes usually involve a single transition-metal atom substituting one carbon atom on the fullerene surface [20] , [21] , [22] . The incorporation of multiple metal atoms on the borospherene surface is due to the flexibility of the 2D boron network, which is a direct result of the electron deficiency of boron. It is interesting to note that the crystal structure of a Ni–Zn boride (Ni 21 Zn 2 B 24 ) was shown to contain characteristic cages of B 20 units, with an octahedral Ni 6 cluster nested inside [35] . Our observation of the Ln 3 B 18 – metallo-borospherenes represents the first isolated molecules of Ln–B cages in the gas phase. To understand the stability of these remarkable cage structures, we carried out fragment MO analyses by first considering the construction of the B 18 framework in two different pathways and then its bonding with the three La atoms, as schematically shown in Fig. 5 . 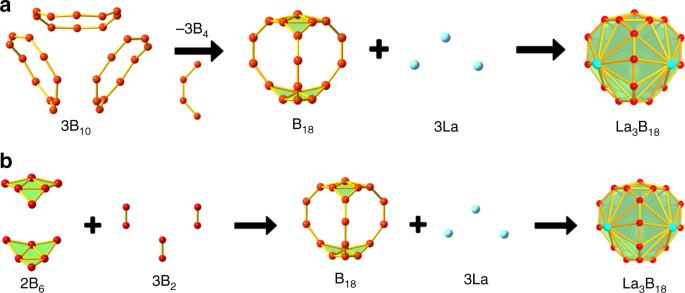Fig. 5: Schematic pathways for the formation of theD3hLn3B18–metallo-borospherenes. Two pathways for the construction of the B18framework and its bonding with the three Ln atoms are depicted.aThe fused B10ring pathway.bThe B2-linked triangular B6pathway. Figure 5a shows one possible path to construct the B 18 framework by the fusion of three B 10 rings. Four of the boron atoms in each B 10 ring are shared with the other B 10 rings, which each coordinate to a La atom to form three shared La©B 10 units. This hypothetical formation pathway of La 3 B 18 – can be expressed by the following steps: 
    3B_10→B_18 + 3B_4    Δ E_1 = 120.1 kcal mol^ - 1
 (1) 
    B_18 + 3La→La_3B_18    Δ E_2 = - 655.8 kcal mol^ - 1
 (2) 
    La_3B_18 + e^- →La_3B_18^-    Δ E_3 = - 68.8 kcal mol^ - 1
 (3) 
    3B_10 + 3La + e^- → 3B_4 + La_3B_18^-   Δ E_A = - 604.5 kcal mol^ - 1
 (4) Fig. 5: Schematic pathways for the formation of the D 3 h Ln 3 B 18 – metallo-borospherenes. Two pathways for the construction of the B 18 framework and its bonding with the three Ln atoms are depicted. a The fused B 10 ring pathway. b The B 2 -linked triangular B 6 pathway. Full size image The energetics were calculated from single-point energy differences of the reactants and products, using the geometries directly taken from the optimized La 3 B 18 – cage at the PBE/TZP level of theory. The interactions between the B 18 framework and the three La atoms are extremely strong (steps 2 and 3), which underlies the stability of the La 3 B 18 – cage. It should be noted that in platonic solids four surfaces are the minimum number to form a 3D object, i.e., the tetrahedron. However, Fig. 5a shows that three La©B 10 surfaces are fused together to form the D 3 h La 3 B 18 – cage. This is because the La©B 10 surface is curved. It turns out that the Ln 3 B 18 – metallo-borospherenes belong to a class of geometry mathematically known as n -gonal hosohedron, which is basically a tessellation of lunes on a spherical surface, such that each lune shares the same two vertices. Thus, the D 3 h La 3 B 18 – cage is a trigonal hosohedron, also known as spherical trihedron, where the two vertices consist of the triangular B 6 units. To the best of our knowledge, such a geometry has not been observed in any cluster or molecular systems heretofore. Figure 5b shows another pathway to construct the La 3 B 18 – cage, in which the B 18 framework is formed by two triangular B 6 motifs linked by three B 2 bridges, such that three B 10 rings are created. This hypothetical pathway can be represented by the following steps: 
    2B_6 + 3B_2 →B_18    Δ E_5 = - 707.9 kcal mol^ - 1
 (5) 
    B_18 + 3La→La_3B_18    Δ E_6 = - 655.8 kcal mol^ - 1
 (6) 
    La_3B_18 + e^- →La_3B_18^-    Δ E_7 = - 68.8 kcal mol^ - 1
 (7) 
    2B_6 + 3B_2 + 3La + e^- →La_3B_18^-    Δ E_B = - 1432.5 kcal mol^ - 1
 (8) The interactions between the B 18 framework and the three La atoms to form the La 3 B 18 – cage are represented by steps 2/3 or 6/7 with an estimated binding energy of 724.6 kcal mol -1 , i.e., 241.5 kcal mol −1 for the binding energy between each La atom and the B 10 ring. This huge La-B 10 binding energy underlies the extraordinary stability of the La 3 B 18 – metallo-borospherene. Compared with the pathway in Fig. 5a , the pathway in Fig. 5b is more favorable energetically since each step is exothermic. We should emphasize, though, that these exercises provide different views of the unprecedented hollow cage structures. The two pathways to construct the La 3 B 18 – cage depicted in Fig. 5 certainly do not represent the mechanisms about how it is formed. The nature of the bonding between B 18 and the La atoms Since the global minimum of B 18 is a planar structure [36] , the stabilization of the 3D B 18 framework is entirely due to its strong bonding with the three La atoms, as discussed above. We have analyzed the nature of the La–B 10 bonding in the La 3 B 18 – metallo-borospherene using several different methods. The MO energy-level diagram and the relevant MOs of La 3 B 18 – derived from the La 3 – and B 18 moieties are shown in Fig. 4 . The 5 e ′′, 9 e ′, and 1 a 1 ′′ MOs of La 3 B 18 – (red-colored) represent the bonding orbitals between the three La atoms and the B 18 moiety, mainly corresponding to the interactions between the irreducible representations, 4 e ′′, 6 e ′, and 1 a 1 ′′ on the B 18 moiety and 6 e ′′, 12 e ′, and 2 a 1 ′′ on the La 3 – moiety (the red highlighted MOs). Supplementary Table S5 gives the compositions of the 5 e ′′, 9 e ′, and 1 a 1 ′′ MOs, which are dominated by contributions from the B 18 moiety. Hence, there is a strong charge transfer from La to B 18 , resulting in a closed-shell La 3 B 18 – with a large HOMO-LUMO gap of 1.51 eV computed at the PBE/TZP level. The La atoms are in their favorite +III oxidation state in La 3 B 18 – , which can be viewed approximately as (La 3+ ) 3 [B 18 10– ]. As shown in Fig. 4 , the 6 e ′′, 12 e ′, and 2 a 1 ′′ irreducible representations on the La 3 – moiety are of La 5 d characters, while the 4 e ′′, 6 e ′, and 1 a 1 ′′ irreducible representations on the B 18 framework are of B 2 p characters. Hence, the 5 e ′′, 9 e ′, and 1 a 1 ′′ MOs also represent significant La 5 d and B 18 2 p covalent bonding. It is the strong covalent and ionic bonding between the La atoms and the B 10 rings that gives rise to the extraordinary stability of the La 3 B 18 – cage structure. These bonding characteristics are found in all lanthanide boride compounds due to the low electronegativity of the lanthanide elements and their diffuse 5 d orbitals [37] . The La–B 10 interactions can be further characterized using the EDA-NOCV method with B 18 (…6 a 1 ′ 2 1 a 1 ′′ 0 6 e ′ 0 4 e ′′ 0 ) and La 3 – (…6 e ′′ 4 2 a 1 ′′ 2 12 e ′ 4 ) fragments, a powerful energy decomposition tool to give insight into chemical bonding [38] . We analyzed the B 18 …La 3 – interaction by the decomposition of the orbital terms into pairwise contributions, as shown in Supplementary Fig. 6 . There are three major terms Δ E 1 , Δ E 2 , and Δ E 3 associated with the deformation densities Δ ρ 1 , Δ ρ 3 , and Δ ρ 3 , respectively. The remaining terms contribute <10% to the total orbital interactions. The color code of the deformation densities indicates the direction of the charge flow from red → blue. It is interesting to see that the 1 a 1 ′′ orbital of La 3 B 18 – , which is analogous to the ( d–p ) δ bonding MO in the Ln 2 B 8 – inverse sandwich complexes [31] , [32] , contributes significantly (25.7% from the EDA-NOCV analyses, Supplementary Fig. 6 ) to the stability of the orbital interaction. The other two stronger Δ ρ 2 (34.8%) and Δ ρ 3 (28.9%) deformation densities correspond to the degenerate 9 e ′ and 5 e ′′ MOs, respectively. The direction of the charge flow is from the La 3 – to the B 18 moiety, consistent with the fragment MO analyses discussed above (Fig. 4 ). We further analyzed the chemical bonding in the La 3 B 18 – metallo-borospherene using the adaptive natural density partitioning (AdNDP) approach [39] , as shown in Fig. 6 . The first row displays nine localized two-center two-electron (2c–2e) σ bonds formed within the three B 2 units and between the B 2 units and the three apexes of the two B 6 triangles. The second row reveals the delocalized bonds in the B 6 triangles, with four three-center two-electron (3c–2e) σ bonds within each B 6 unit. The multi-center 12c–2e and 18c–2e delocalized bonds can be viewed as π bonds within the B 6 units. The third row represents totally delocalized σ and π bonds within the B 18 framework. The last row shows five totally delocalized 21c–2e bonds between the La atoms and the B 18 framework, corresponding to the 5 e ′′, 9 e ′, and 1 a 1 ′′ MOs in Fig. 4 . 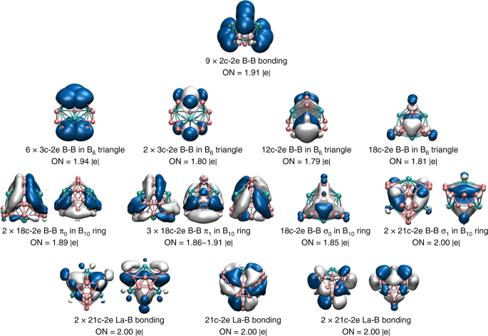Fig. 6: Chemical bonding analyses of La3B18–(D3h1A1). The analyses were done using the AdNDP method29. ON stands for occupation number. We also found that the La 3 B 18 – metallo-borospherene possesses both 3D aromaticity with calculated nucleus-independent chemical shifts (NICS) [40] of −47.87 ppm at the cage center, and planar aromaticity on each B 6 triangles with NICS(0) of −31.44 ppm and NICS(1) of −2.16 above the plane center, as shown in Supplementary Table 6 , where the aromaticity in the metallo-borospherene is compared with that of the recently synthesized cubic [Zn I ] 8 compound [41] . Fig. 6: Chemical bonding analyses of La 3 B 18 – ( D 3 h 1 A 1 ). The analyses were done using the AdNDP method [29] . ON stands for occupation number. Full size image We also performed bond-order index analyses for the B–B and La–B interactions, as presented in Supplementary Table 7 . The B 2 bridges have shorter bond lengths and higher bond orders than those of the B 6 triangles. In terms of the La–B interactions, the distances and bond order indices are similar to those in the lanthanide–boron complexes reported previously [30] , [31] , [32] , [33] . A new class of spherical trihedron metallo-borospherenes The discoveries of the La 3 B 18 – and Tb 3 B 18 – metallo-borospherenes suggest that other lanthanide elements could also form similar structures because of the similarity in the chemical properties of the whole series of lanthanides. We have calculated the D 3 h cage structures for all the lanthanide elements, Ln 3 B 18 – (Ln = Ce–Lu). The coordinates obtained at the PBE0 level are given as Supplementary Data 1 , whereas those of La 3 B 18 – and La 3 B 18 are provided in Supplementary Table 8 . All these structures are indeed minima on their potential energy surfaces. Hence, we conclude that there indeed exist a whole class of Ln 3 B 18 – metallo-borospherenes. While borospherenes have not been observed beyond the B 40 cluster [42] , the unique bonding characteristics between lanthanide and boron suggest that other lanthanide metallo-borospherenes with different sizes and Ln x B y – stoichiometries may exist. Recent studies of transition-metal borides showed that the metal–boron interactions have major influences on their magnetic properties [43] , [44] . Hence, the understanding of Ln–B interactions in the metallo-borospherene systems may provide insights for the design of lanthanide borides with tunable magnetic or catalytic properties. In conclusion, we report the observation of the first tri-lanthanide-doped boron cage clusters (metallo-borospherenes), in which the metal atoms are integral parts of the cage surface. Photoelectron spectra of two representative systems, Ln 3 B 18 – (Ln = La, Tb), show similar and relatively simple spectral patterns, suggesting that they have similar highly symmetric structures. Theoretical calculations reveal that the Ln 3 B 18 – anions have cage-like structures with D 3 h symmetry: two planar B 6 triangular units linked by three B 2 bridges to form the B 18 framework consisting of three shared B 10 rings coordinated to the three Ln atoms. Strong ionic and covalent chemical bonding is found between the Ln atoms and the B 18 framework. The extraordinary stabilities of the metallo-borospherenes are understood by various theoretical analyses. La 3 B 18 – is found to have a closed-shell electron configuration with a large HOMO-LUMO gap and possesses 3D aromaticity. The Ln 3 B 18 – cage complexes are expected to exist for all lanthanide elements, suggesting the possibility that there may exist a large class of lanthanide metallo-borospherenes with different Ln/B stoichiometries and tunable properties. Experimental details The experiments were carried out using a magnetic-bottle PES apparatus equipped with a laser vaporization supersonic cluster source, details of which have been published elsewhere [11] . The La 3 B 18 – and Tb 3 B 18 – clusters were produced by laser vaporization of a La/ 11 B or Tb/ 11 B mixed target, respectively. The laser-induced plasma was cooled by a He carrier gas seeded with 5% Ar, initiating nucleation between the boron and lanthanide atoms. The nascent clusters were entrained in the carrier gas and underwent a supersonic expansion. Negatively-charged clusters were extracted from the collimated cluster beam and analyzed by a time-of-flight mass spectrometer. Both pure (B n – ) and mixed (Ln x B y – ) clusters were produced from the cluster source. The La 3 B 18 – and Tb 3 B 18 – clusters of current interest were mass-selected and photodetached by the 193 nm (6.424 eV) radiation from an ArF excimer laser or the fourth harmonics from a Nd:YAG laser (266 nm, 4.661 eV). Photoelectrons were collected and analyzed in a 3.5-m-long electron flight tube at nearly 100% efficiency. The photoelectron spectra were calibrated by the known transitions of Au – and Bi – . The resolution of the PES apparatus (ΔKE/KE) was around 2.5%, that is, about 25 meV for photoelectrons with 1 eV kinetic energy (KE). Computational methods Unbiased global-minimum structural searches for the La 3 B 18 – cluster were performed using the TGMin 2.0 code [45] . The global minimum structure of Tb 3 B 18 – was not searched separately. More than 2000 structures were evaluated for La 3 B 18 – using the constrained Basin–Hopping algorithm at the PBE/DZP [46] , [47] level from the ADF 2017 software [48] . A D 3 h cage structure was found to be the global minimum, which was significantly lower in energy in comparison to the next lowest-lying isomer (Supplementary Fig. 2 ). To confirm the stability of the global minimum, we conducted another 500 structural searches, using the D 3 h cage as the seed structure. No structures with lower energies were found. All the local minima were verified via harmonic vibrational frequency calculations. The frozen-core approximation was employed for the inner shells of [1 s 2 ] for B and [1 s 2 −4 d 10 ] for the La atoms. The zero-order regular approximation [49] was applied, to account for the scalar relativistic effects. Low-lying isomers were subsequently optimized using the PBE and PBE0 density functionals [50] along with the TZP basis sets. Born–Oppenheimer molecular dynamic simulations were further carried out on La 3 B 18 – for 13 ps using the CP2K code [51] at different temperatures, from 300 to 1000 K (Supplementary Fig. 4 ). To minimize the 4 f -electron induced complexity (i.e. spin multiplicity) and considering the negligible geometry change due to the occupations of the localized 4 f orbitals (radial-density maximum probability radii <0.5 Å), we used the 4 f -in-core pseudopotentials [34] for the lanthanide elements to optimize the geometric parameters in the other Ln 3 B 18 – (Ln = Ce–Lu) species. The simulation of the PE spectra was done using the ΔSCF-TDDFT method [52] with the SAOP exchange-correlation functional [53] to account for the long-range interactions. The ground state adiabatic and vertical detachment energies were calculated at the DFT levels, as well as the more accurate DLPNO-CCSD(T) level [54] with the Def2-TZVP basis sets [55] and the Def2-TZVPP pseudopotential for La [34] , utilizing the AutoAux generation procedure [55] . We also used the 4 f -in-core pseudopotential [34] for the simulation of the PE spectrum of Tb 3 B 18 – without consideration of the 4 f electron detachment channels. Previous studies showed that such detachment channels carried very low detachment cross sections at the low detachment photon energies used and the main PES features of Ln–B binary clusters were dominated by MOs with Ln sd or B sp characters [31] , [32] , [33] . Chemical bonding and electronic structure analyses were carried out by canonical molecular orbital (MO) theory and the semi-localized AdNDP method [39] . We also performed calculations using the energy decomposition analysis–natural orbitals for chemical valence (EDA–NOCV) approach [38] to quantitatively elucidate the bonding mechanisms between the B 18 and La 3 – moieties. The bond order indexes of different interatomic interactions were calculated using the Mayer [56] , Gopinathan–Jug (G–J) [57] , and Nalewajski–Mrozek schemes [58] .